Alternatively activated macrophages promote pancreatic fibrosis in chronic pancreatitis Chronic pancreatitis (CP) is a progressive and irreversible inflammatory and fibrotic disease with no cure. Unlike acute pancreatitis (AP), we find that alternatively activated macrophages (AAMs) are dominant in mouse and human CP. AAMs are dependent on interleukin (IL)-4 and IL-13 signalling, and we show that mice lacking IL-4Rα, myeloid-specific IL-4Rα and IL-4/IL-13 were less susceptible to pancreatic fibrosis. Furthermore, we demonstrate that mouse and human pancreatic stellate cells (PSCs) are a source of IL-4/IL-13. Notably, we show that pharmacologic inhibition of IL-4/IL-13 in human ex vivo studies as well as in established mouse CP decreases pancreatic AAMs and fibrosis. We identify a critical role for macrophages in pancreatic fibrosis and in turn PSCs as important inducers of macrophage-alternative activation. Our study challenges and identifies pathways involved in crosstalk between macrophages and PSCs that can be targeted to reverse or halt pancreatic fibrosis progression. Chronic pancreatitis (CP) is characterized by progressive and what is thought to be irreversible damage to the pancreas, with end result of endocrine and exocrine insufficiency [1] . CP histologic features include chronic inflammation, fibrosis, acinar cell atrophy and distorted and/or blocked ducts [2] , [3] . The management of CP is challenging with focus on the management of complications, and most patients remain symptomatic despite limited supportive therapy. Currently, there are no effective methods to limit progression or reverse this syndrome [4] . Recurrent AP or pancreatic insults lead to necroinflammation and are linked to the development of pancreatic fibrosis (the necrosis–fibrosis concept) [4] . Recent in vitro and in vivo studies demonstrate the central role of activated pancreatic stellate cells (PSCs) in CP-associated fibrogenesis by regulating the synthesis and degradation of extracellular matrix proteins [5] , [6] . PSCs are activated by many factors such as toxic factors associated with pancreatitis (for example, ethanol) and/or by cytokines released from injured acinar cells and/or pancreas-infiltrating leukocytes (such as macrophages and neutrophils) [7] . Macrophages are innate immune cells, which are for simplicity divided into two spectra of major types based on Siamon Gordon’s scheme: (1) classically activated macrophages (M1), induced by interferon gamma (IFNγ) and/or lipopolysaccharide, characterized by the production of reactive oxygen and nitrogen species and thought to play a critical role in host defense and antitumour immunity; and (2) alternatively activated macrophages (AAMs, M2), on exposure to IL-4/IL-13, are characterized by cell surface expression of scavenger receptors CD206. AAMs play key roles in dampening inflammation, promote wound-healing, fibrosis and tumorigenesis [8] . Recent studies highlighted the function of macrophages as master regulators of fibrosis [9] . Distinct macrophage populations contribute important activities towards the initiation, maintenance and resolution phase of fibrosis [9] , [10] . Macrophages have been observed in close proximity to PSCs in human pancreatic fibrosis, and their presence observed in rat model of CP, although not well defined, their potential role in CP has been suggested [11] , [12] . Thus, the mechanism(s) by which crosstalk between activated stellate cells and macrophages trigger and sustain the fibrotic process during CP is not known. Delineating immune responses involved in the fibrotic processes will improve our understanding of disease pathogenesis and allow for designing novel therapeutics that can either treat and/or reverse the disease. Our study investigates and identifies macrophage characteristics and function in CP. In this study, we demonstrate that progression to CP is associated with alternative activation of macrophages and show an important role for the IL-4/IL-13 pathway in a crosstalk between macrophages and PSCs using in vivo and in vitro animal studies as well as ex vivo human primary cells. Notably, blocking IL-4/IL-13 using a peptide antagonist we show a therapeutic effect in established experimental CP and proof-of-concept therapeutic ex vivo effect using human samples. These studies are likely to offer potential benefit in a disease for which currently no active therapeutic agent exists and as such the disease is deemed progressive and irreversible. Macrophages are increased in mouse and human CP Studies on pathogenic mechanism of fibrosis in human CP are restricted by limited availability of tissues obtained from surgery. Therefore, animal models, despite their limitation in recapitulating all aspects of human disease, have been useful to investigate the initiation and progression of CP [13] , [14] . In mice, hyperstimulation of the pancreas with cholecystokinin analogue caerulein leads to AP, and continuous acute injury to the pancreas drives chronic inflammation of the pancreas [4] , [14] . To generate experimental CP, we induced AP in a repetitive manner over 4 weeks (three times per week). Mice undergoing repetitive treatment with caerulein revealed morphologic signs of CP with leukocyte infiltration, pancreatic fibrosis and acinar cell loss corresponding to small size of the pancreas relative to body weight ( Supplementary Fig. 1a–c ). We next sought to investigate the immune responses in experimental CP. Using Luminex assay, we compared multiple cytokine and chemokine expression profiles in the pancreas from control and CP mice. As expected, the profibrotic cytokine, transforming growth factor beta (TGFβ) was increased in the pancreas of CP mice. However, pro-inflammatory cytokines (IL-1β and IL-6), which are known to be increased during acute inflammation, were downregulated in CP. Chronic repeated caerulein administration and pancreas harvest 3 days after the last injection is consistent with the development of a chronic and not AP. Furthermore, macrophage-associated cytokines and chemokines (granulocyte–macrophage CSF, granulocyte CSF, chemokine (C-C motif) ligand (CCL)2/monocyte-specific chemokine(MCP)-1, CCL7/MCP-3 and CCL3/macrophage inflammatory protein (MIP)1A) were upregulated, suggesting that monocytes/macrophages play an important role during CP. In contrast, no significant increase in CXCL1, a neutrophil chemoattractant with role in AP [15] , was observed ( Fig. 1a ). 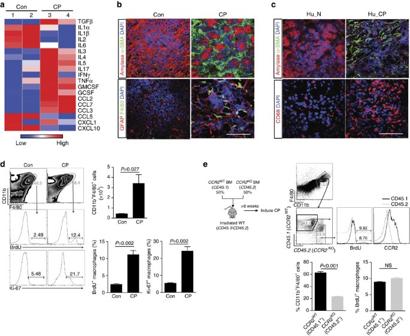Figure 1: Macrophages are increased in mouse and human CP. (a) Heat map of cytokine and chemokine expressions in the pancreas lysates from control (Con) and CP mice quantitated via the Luminex analysis. (b) Representative immunofluorescence images of the pancreas from control and CP mice stained with amylase (acinar cells), α-SMA and GFAP (PSCs), F4/80 (macrophages) and 4,6-diamidino-2-phenylindole (DAPI). Scale bars, 50 μm. (c) Representative immunofluorescence images of the human pancreas from paired normal and CP tissue stained with amylase, α-SMA, CD68 (macrophages) and DAPI. Scale bars, 50 μm. (d) Pancreatic leukocytes were isolated from control and CP mice and analysed using flow cytometry for macrophages (gated on CD45.2+cells first as shown inSupplementary Fig. 3, then CD11b+F4/80+) numbers, BrdU incorporation, Ki-67 expression (n⩾3 per group). (e)CCR2WTCD45.1+CD45.2+C57BL/6 mice were lethally irradiated and reconstituted with a 1:1 mixture of BM cells fromCCR2WTCD45.1+andCCR2KOCD45.2+mice over 8 weeks. Mice were injected with caerulein to induce CP as described in the Methods section, and macrophages (gated on CD11b+F4/80+without prior CD45.2 gating) were analysed using flow cytometry following pancreatic leukocyte isolation. Representative flow cytometry plots and bar graphs depicting the proportion of macrophages and BrdU incorporation originating fromCCR2WTCD45.1+(black line) versus fromCCR2KOCD45.2+(grey line) and CCR2 expression are shown.n=3 for each group; mean±s.e.m., ns, not significant (unpaired two-tailed Student’st-test). Figure 1: Macrophages are increased in mouse and human CP. ( a ) Heat map of cytokine and chemokine expressions in the pancreas lysates from control (Con) and CP mice quantitated via the Luminex analysis. ( b ) Representative immunofluorescence images of the pancreas from control and CP mice stained with amylase (acinar cells), α-SMA and GFAP (PSCs), F4/80 (macrophages) and 4,6-diamidino-2-phenylindole (DAPI). Scale bars, 50 μm. ( c ) Representative immunofluorescence images of the human pancreas from paired normal and CP tissue stained with amylase, α-SMA, CD68 (macrophages) and DAPI. Scale bars, 50 μm. ( d ) Pancreatic leukocytes were isolated from control and CP mice and analysed using flow cytometry for macrophages (gated on CD45.2 + cells first as shown in Supplementary Fig. 3 , then CD11b + F4/80 + ) numbers, BrdU incorporation, Ki-67 expression ( n ⩾ 3 per group). ( e ) CCR2 WT CD45.1 + CD45.2 + C57BL/6 mice were lethally irradiated and reconstituted with a 1:1 mixture of BM cells from CCR2 WT CD45.1 + and CCR2 KO CD45.2 + mice over 8 weeks. Mice were injected with caerulein to induce CP as described in the Methods section, and macrophages (gated on CD11b + F4/80 + without prior CD45.2 gating) were analysed using flow cytometry following pancreatic leukocyte isolation. Representative flow cytometry plots and bar graphs depicting the proportion of macrophages and BrdU incorporation originating from CCR2 WT CD45.1 + (black line) versus from CCR2 KO CD45.2 + (grey line) and CCR2 expression are shown. n =3 for each group; mean±s.e.m., ns, not significant (unpaired two-tailed Student’s t -test). Full size image To understand the relevance of these observations to human CP, we compared them with normal pancreas tissue sections. Immunofluorescence analysis showed that CD68 + macrophages were increased in human CP ( Fig. 1c ). A similar trend was observed in mice; macrophage marker F4/80 analysis revealed that macrophages are abundant in CP as compared with the normal pancreas of mice ( Fig. 1b ). Furthermore, the number of pancreatic macrophages (CD11b + F4/80 + ) analysed using flow cytometry was markedly increased in CP mice ( Fig. 1d ). Macrophage tissue infiltration occurs in two distinct ways: recruitment of monocyte precursors and proliferation of resident cells [16] . We used Ki-67 expression and 5-bromodeoxyuridine (BrdU) incorporation to determine the proportion of proliferating macrophages. We found that BrdU + and Ki-67 + macrophages were both increased in CP mice accounting for ∼ 12–25% of the pancreatic macrophages ( Fig. 1d ), indicating proliferation of either resident macrophages or recruited monocytes that differentiated to macrophage contributed to some of the macrophage accumulation in CP. During AP, monocytes are attracted to the injured pancreas before their differentiation into macrophages in a CCR2-dependent manner [17] , [18] . CCR2 ligands such as CCL2 (MCP-1) and CCL7 (MCP-3) are also elevated in CP ( Fig. 1a ). Considering that the model of CP is based on repetitive acute injury, we hypothesized that, in addition to proliferation, a significant proportion of macrophages in CP arises from monocyte recruitment. To confirm this hypothesis, we set up a competitive bone marrow (BM) chimera by lethally irradiating recipient CCR2 WT CD45.1 + CD45.2 + C57BL/6 mice and reconstituting them with a 1:1 mixture of BM derived from CCR2 wild-type (WT; CCR2 WT CD45.1 + ) and CCR2 knockout ( CCR2 KO CD45.2 + ) mice so that macrophages derived from CCR2 KO and CCR2 WT mice could be distinguished from one another as well as from those of the recipient mice based on the allotypic CD45 markers. Following 8 weeks of engraftment and induction of CP, we found that the number of CCR2 WT macrophages greatly outnumbered CCR2 KO macrophages. However, there was no difference in proliferation (BrdU incorporation) observed between CCR2 WT and CCR2 KO cells, supporting CCR2’s role in monocyte recruitment as a significant contributor to macrophage accumulation in CP ( Fig. 1e ). To further confirm our findings, we induced CP in nonirradiated wild-type ( CCR2 WT ) and CCR2 knockout ( CCR2 KO ) mice. As shown in Supplementary Fig. 2 , CCR2 deficiency limits pancreatic macrophage accumulation in CP, and no proliferation difference is observed between presence and absence of CCR2, which is consistent with the above BM chimera findings. However, in the absence of CCR2 there is still monocyte/macrophage recruitment to the pancreas during CP, suggesting that CCR2-independent mechanism(s) also exist. Thus, both monocyte recruitment (via CCR2-dependent and -independent mechanisms) and macrophage proliferation account for macrophage accumulation during CP progression. AAMs are dominant in mouse and human CP In order to determine the polarization state of macrophages in CP, SSC-A low CD11b + monocytes/macrophages were sorted from both control and CP mice for gene expression analysis. Sorting strategy and purity of monocytes/macrophages are shown in Supplementary Fig. 3 . Gene expression profile revealed an increase in M2-associated genes, such as YM1 , CD206 , CD301 , IL-10 , TGFβ , and PDGFβ , in pancreatic monocytes/macrophages of CP as compared with controls ( Fig. 2a ). Moreover, the presence of AAMs in CP was further verified using flow cytometry as shown by increased M2-associated markers (CD206, IL-10 and IL-4Rα), and decreased or unchanged expression of M1-associated markers (major histocompatibility complex class II (MHCII) and tumour-necrosis factor alpha (TNFα); Fig. 2b ). In contrast, by assessing dynamic gene expression of pancreatic macrophages during AP induction, classical activation profile with increased TNFα and decreased CD206, CD301 was found in AP mice ( Supplementary Fig. 4a,b ). Unlike TNFα, IL-10 expression can be seen as late response in M1s (ref. 19 ), which is consistent with our AP data ( Supplementary Fig. 4a ). Nevertheless, IL-10 in AP is expressed at much lower level as compared with CP in pancreatic macrophages ( Fig. 2 ), although not to the same extent, slightly higher level of YM1 expression is seen in CP as compared with AP. Arg1 has recently been shown to be expressed by both classic and AAMs [20] . Flow cytometric data were consistent with the histologic analysis of pancreas from CP mice on the basis of immunofluorescence staining where a majority of F4/80 + macrophages were positive for CD206 but not TNFα. Similar findings were observed in human CP tissues, where CD68 + cells expressed CD206, but not TNFα ( Fig. 2c,d ). 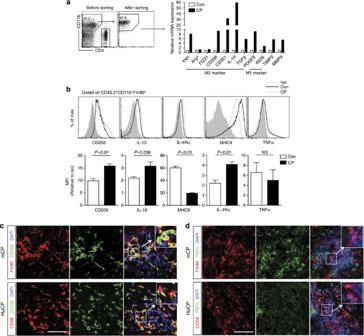Figure 2: Alternatively activated macrophages are dominant in mouse and human CP. (a) Pancreatic leukocytes from control and CP mice were isolated and sorted for SSC-AlowCD11b+monocytes/macrophages (five mice were pooled for each group). Markers of alternatively and classically activated macrophages were assessed using quantitative PCR. Expression of the genes was normalized to their relative expression in control mice. (b) Expression of alternative activation markers (CD206, IL-10 and IL-4Rα) and classical activation markers (MHCII and TNFα) in pancreatic macrophages of indicated mice were monitored using flow cytometry. MFI, mean fluorescence intensity; data presented as mean± s.e.m. (unpaired two-tailed Student’st-test). (c) Representative immunofluorescence images of mouse and human CP tissues co-stained with macrophage F4/80 (mouse) or CD68 (human), CD206 (M2 marker) and DAPI (nuclei). (d) Representative immunofluorescence images of mouse and human CP tissues, co-stained with F4/80 or CD68, TNFα (M1 marker) and DAPI. Scale bars, 50 μm. Figure 2: Alternatively activated macrophages are dominant in mouse and human CP. ( a ) Pancreatic leukocytes from control and CP mice were isolated and sorted for SSC-A low CD11b + monocytes/macrophages (five mice were pooled for each group). Markers of alternatively and classically activated macrophages were assessed using quantitative PCR. Expression of the genes was normalized to their relative expression in control mice. ( b ) Expression of alternative activation markers (CD206, IL-10 and IL-4Rα) and classical activation markers (MHCII and TNFα) in pancreatic macrophages of indicated mice were monitored using flow cytometry. MFI, mean fluorescence intensity; data presented as mean± s.e.m. (unpaired two-tailed Student’s t -test). ( c ) Representative immunofluorescence images of mouse and human CP tissues co-stained with macrophage F4/80 (mouse) or CD68 (human), CD206 (M2 marker) and DAPI (nuclei). ( d ) Representative immunofluorescence images of mouse and human CP tissues, co-stained with F4/80 or CD68, TNFα (M1 marker) and DAPI. Scale bars, 50 μm. Full size image PSCs promote alternative activation of macrophages Macrophages are highly heterogeneous cells that can rapidly change their activation status and function in response to local microenvironment signals [21] , [22] . In light of the crucial role played by PSCs in CP, we asked whether PSCs might contribute to macrophage polarization and function. We isolated PSCs from CP mice and assessed their cytokine production with the Luminex assay. Overall, the expression of several pro-inflammatory cytokines such as IFNγ, TNFα and IL-1β was very low. In contrast, PSCs secreted higher levels of IL-4, IL-5, IL-13, IL-10 and TGFβ, indicating a Th2 and profibrogenic cytokine bias ( Fig. 3a ). 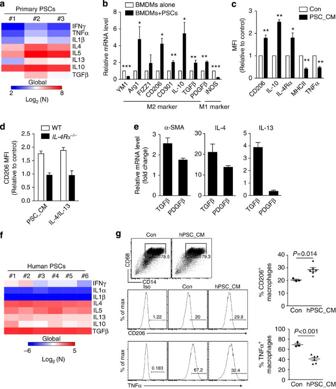Figure 3: Mouse and human pancreatic stellate cells promote alternative macrophage polarization. (a) Culture supernatants from primary PSCs isolated from CP mice were collected and quantitated via the Luminex analysis, cytokine data presented as a heat map. (b) Analysis of macrophage activation-associated genes in BMDMs cocultured in the presence or absence of PSCs for 2 days. Bar graphs represent BMDM gene expression in the presence of PSCs relative to absence of PSCs (BMDMs alone). (c) BMDMs were cultured with PSC conditioned medium (PSC_CM) or control medium (Con) for 24 h, and expression of CD206, IL-10, IL-4Rα, MHCII and TNFα determined using flow cytometry. (d) BMDMs from WT orIL-4Rα−/−mice were cultured with PSC_CM or IL-4/IL-13 (as a positive control for alternative macrophage polarization) for 24 h, and the expression of CD206 was examined using flow cytometry. (e) Mouse PSCs were cultured with TGFβ (5 ng ml−1), PDGFβ (10 ng ml−1) or controls for 6 h and indicated gene expression was determined using qPCR. Representative bar graphs show relative mRNA expression over control treatments. (f) Culture supernatants from primary PSCs derived from PDAC pieces (nos 2, 4, 6), normal margin of patients with PDAC (nos 3 and 5) and normal pancreas (no. 1; patient with nonpancreatic tumour requiring partial resection of the pancreas) were collected and quantitated via the Luminex analysis. Data presented as a cytokine heat map expression. (f) Monocyte-derived human macrophages were exposed to the conditioned medium from human PSCs (hPSC_CM) for 24 h. The expressions of CD206 and TNFα were examined using flow cytometry. *P<0.05, **P<0.01, ***P<0.001. Data presented as means±s.e.m. (unpaired two-tailed Student’st-test). Figure 3: Mouse and human pancreatic stellate cells promote alternative macrophage polarization. ( a ) Culture supernatants from primary PSCs isolated from CP mice were collected and quantitated via the Luminex analysis, cytokine data presented as a heat map. ( b ) Analysis of macrophage activation-associated genes in BMDMs cocultured in the presence or absence of PSCs for 2 days. Bar graphs represent BMDM gene expression in the presence of PSCs relative to absence of PSCs (BMDMs alone). ( c ) BMDMs were cultured with PSC conditioned medium (PSC_CM) or control medium (Con) for 24 h, and expression of CD206, IL-10, IL-4Rα, MHCII and TNFα determined using flow cytometry. ( d ) BMDMs from WT or IL-4Rα −/− mice were cultured with PSC_CM or IL-4/IL-13 (as a positive control for alternative macrophage polarization) for 24 h, and the expression of CD206 was examined using flow cytometry. ( e ) Mouse PSCs were cultured with TGFβ (5 ng ml −1 ), PDGFβ (10 ng ml −1 ) or controls for 6 h and indicated gene expression was determined using qPCR. Representative bar graphs show relative mRNA expression over control treatments. ( f ) Culture supernatants from primary PSCs derived from PDAC pieces (nos 2, 4, 6), normal margin of patients with PDAC (nos 3 and 5) and normal pancreas (no. 1; patient with nonpancreatic tumour requiring partial resection of the pancreas) were collected and quantitated via the Luminex analysis. Data presented as a cytokine heat map expression. ( f ) Monocyte-derived human macrophages were exposed to the conditioned medium from human PSCs (hPSC_CM) for 24 h. The expressions of CD206 and TNFα were examined using flow cytometry. * P <0.05, ** P <0.01, *** P <0.001. Data presented as means±s.e.m. (unpaired two-tailed Student’s t -test). Full size image To explore whether factors released by PSCs have the ability to change the activation and polarization status of pancreatic macrophages, we cocultured BM-derived macrophages (BMDMs) with the PSCs in vitro . BMDMs after being cocultured with activated PSCs exhibited alternative activation (M2) profile with increased CD206, CD301, IL-10, TGFβ and PDGFβ mRNA expression but had decreased expression of inducible nitric oxide synthase (M1 marker; Fig. 3b ). Moreover, conditioned medium from the PSCs resulted in upregulation of CD206, IL-10 and IL-4Rα, and downregulation of MHCII and TNFα expression ( Fig. 3c ), suggesting that factors released by PSCs promoted macrophage polarization towards M2. Th2 cytokines such as IL-4/IL-13 mediate alternate activation of macrophages via IL-4 receptor. Thus, we tested whether the PSC supernatant is mediating M2 polarization via IL-4Rα using BMDMs from WT and IL-4Rα −/− mice. Compared with WT BMDMs, IL-4Rα −/− BMDMs were unable to be alternatively activated by the conditioned medium from the PSCs ( Fig. 3d ). Moreover, PSC conditioned medium was as good as exogenously added IL-4/IL-13, standard M2 polarizing conditions. The macrophages produced TGFβ and PDGFβ ( Fig. 3b ), previously shown to be potent activators of PSCs [6] . To investigate the effect of these factors on PSC-mediated macrophage polarization, we treated PSCs with TGFβ and PDGFβ and examined the expression of IL-4/IL-13. Interestingly, our study shows that PDGFβ and in particular TGFβ were capable not only of inducing alpha smooth muscle actin (α-SMA) but also IL-4 and IL-13 genes in the PSCs ( Fig. 3e ). Taken together, these results suggest that PSCs promote macrophage alternative activation in an IL-4Rα signalling-dependent manner, and the macrophages in turn have the ability to induce PSC activation and produce IL-4R ligands. To further validate our finding in human, we isolated PSCs from six patients (hPSCs) who underwent surgical resection (three from normal pancreas, three from pancreatic cancer) of the pancreas. We confirmed that the cultured cells had a PSC phenotype using immunofluorescence staining of Glial fibrillary acidic protein (GFAP) and α-SMA ( Supplementary Fig. 7a ). Consistent with mouse PSCs, hPSCs secreted relatively higher levels of Th2 as compared wirh Th1 cytokines ( Fig. 3f ). Macrophages derived from circulating monocytes of healthy blood donors were cocultured with supernatant of the hPSCs in an effort to translate the mouse studies. Conditioned medium from all six hPSCs increased CD206, but decreased TNFα expression in the human macrophages, indicating that factors released from hPSCs also promote macrophage polarization towards M2 ( Fig. 3g ). IL-4Rα signal deficiency limits AAMs and protects against CP To investigate the importance of macrophage alternative activation in CP, we induced CP in mice lacking IL-4 and IL-13. IL-4/IL-13 −/− mice have been shown to lack AAMs in other disease models [23] . Unlike WT counterparts, IL-4/IL-13 −/− mice were less susceptible to CP, as shown by the larger relative pancreas size (WT: from 5.95±0.11 to 1.71±0.05; IL-4/IL-13 −/− : from 5.98±0.20 to 2.89±0.07; Fig. 4a ), lower fibrosis-associated gene expression in the pancreas such as αSMA ( α -SMA) and Col1α1 (Collagen1A1) using real-time PCR and immunofluorescence analysis ( Fig. 4b,c ). Moreover, compared with WT mice, macrophages isolated from the IL-4/IL-13 −/− mice pancreas had lower expression of CD206, suggesting a decrease in alternative activation of pancreatic macrophages ( Fig. 4d ). 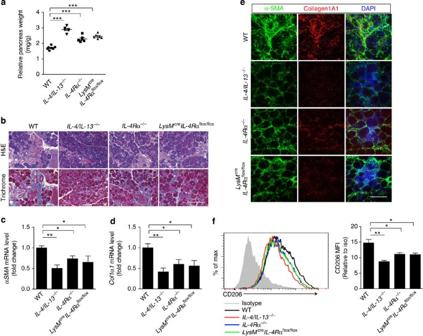Figure 4: Global or myeloid-specific IL-4Rα deficiency is protective against CP. WT,IL-4/IL-13−/−,IL-4Rα−/−andLysMcreIL-4Rαflox/floxmice were subjected to caerulein-induced CP. (a) Relative pancreas weight (pancreas weight/body weight) are shown.n=6–7 per genotype, means±s.e.m., ***P<0.001,ns, not significant,P<0.05 considered significant (one-way analysis of variance (ANOVA), Tukey’spost hoctest). (b) Histologic feature of the pancreas from different genotypes of mice are shown using H&E and Trichrome staining. Scale bar, 200 μm. (c,d) Quantitative RT–PCR analysis of fibrosis-associated genesαSMA(α-SMA) andCol1α1(Collagen1A1) in the pancreas of indicated mice is shown. Means±s.e.m. *P<0.05, **P<0.01,ns, not significant (one-way ANOVA, Tukey’spost hoctest). (e) Representative immunofluorescence images of the pancreas from each genotype of mice are shown (co-stained with α-SMA, Collagen1A1 and DAPI). (f) Flow cytometry analysis of pancreatic macrophages (CD11b+F4/80+) CD206 expression (MFI) from different genotypes of mice is shown. Means±s.e.m., *P<0.05, **P<0.01,ns, not significant (one-way ANOVA, Tukey’spost hoctest). Figure 4: Global or myeloid-specific IL-4Rα deficiency is protective against CP. WT, IL-4/IL-13 −/− , IL-4R α −/− and LysM cre IL-4Rα flox/flox mice were subjected to caerulein-induced CP. ( a ) Relative pancreas weight (pancreas weight/body weight) are shown. n =6–7 per genotype, means±s.e.m., *** P <0.001, ns , not significant, P <0.05 considered significant (one-way analysis of variance (ANOVA), Tukey’s post hoc test). ( b ) Histologic feature of the pancreas from different genotypes of mice are shown using H&E and Trichrome staining. Scale bar, 200 μm. ( c , d ) Quantitative RT–PCR analysis of fibrosis-associated genes αSMA (α-SMA) and Col1α1 (Collagen1A1) in the pancreas of indicated mice is shown. Means±s.e.m. * P <0.05, ** P <0.01, ns , not significant (one-way ANOVA, Tukey’s post hoc test). ( e ) Representative immunofluorescence images of the pancreas from each genotype of mice are shown (co-stained with α-SMA, Collagen1A1 and DAPI). ( f ) Flow cytometry analysis of pancreatic macrophages (CD11b + F4/80 + ) CD206 expression (MFI) from different genotypes of mice is shown. Means±s.e.m., * P <0.05, ** P <0.01, ns , not significant (one-way ANOVA, Tukey’s post hoc test). Full size image To determine whether the observed decrease in pancreatic fibrosis was a direct consequence of IL-4Rα signalling, we used mice with global deletion of IL-4Rα and LysM cre IL-4Rα flox/flox mice, where IL-4Rα is deleted specifically in myeloid cells (i.e., macrophages and neutrophils) [23] , [24] to induce CP. As expected, pancreatic macrophages from IL-4Rα −/− and LysM cre IL-4Rα flox/flox mice displayed impaired alternative activation under chronic inflammation ( Fig. 4f ). IL-4Rα −/− and LysM cre IL-4Rα flox/flox mouse pancreas were less fibrotic and had lower expression of fibrosis-associated markers ( α -SMA and Collengen1A1) as compared with their WT counterparts ( Fig. 4a–e ). Notably, IL-4Rα −/− and LysM cre IL-4Rα flox/flox mice showed no obvious difference in pancreatic fibrosis and alternative macrophage activation, suggesting that the protective effect of IL-4Rα inhibition is mediated via absence of this receptor or signalling on myeloid cells or macrophages. Thus, in this model of CP, AAMs are important contributors to disease pathogenesis. To further confirm an IL-4Rα requirement for macrophage alternative activation in CP, we set up a mixed BM chimera with a 1:1 BM reconstitution from IL-4Rα WT CD45.1 + and IL-4Rα −/− CD45.2 + mice in order to compare IL-4Rα-sufficient and -deficient macrophages in the same environment of CP ( Supplementary Fig. 5a ). In such a competitive environment, CD206 expression in IL-4Rα WT macrophages (CD11b + F4/80 + ) was upregulated following CP induction, whereas no significant difference in CD206 expression was observed in IL-4Rα −/− macrophages ( Supplementary Fig. 5b ). No difference in proliferation between IL-4Rα WT and IL-4Rα −/− pancreatic macrophages was observed ( Supplementary Fig. 5c ). In sum, these findings indicate that IL-4R α signalling in macrophages is in part required for pancreatic macrophage alternative activation and fibrosis during CP development. IL-4/IL-13 blockade ameliorates established CP In light of the above findings and the importance of IL-4Rα signalling in experimental CP-associated fibrogenesis, we wanted to test whether IL-4Rα signalling blockade can be used as a therapy in established disease. We obtained IL-4/IL-13-blocking peptide (a potent cyclic peptide ∼ 1.5 kD) from Dr Murali’s laboratory. We first tested the inhibitor in an in vitro titration assay, and at 1 μM the inhibitor significantly decreased mouse IL-4/IL-13-induced M2 polarization and CD206 expression ( Supplementary Fig. 6 ). We then tested the effect of the inhibitor in mice that were already subjected to repeated caerulein injection for 2 weeks, where significant decrease in pancreas size and α-SMA expression was present ( Supplementary Fig. 1d,e ). Compared with control treatment group, the inhibitor treatment limited pancreas fibrosis ( Fig. 5a–e ). Furthermore, blockade of alternative activation of pancreatic macrophages by the inhibitor was confirmed using flow cytometry ( Fig. 5f ). These observations, as a proof-of-concept, demonstrate potential for treating CP. We then tested the inhibitor’s ability in blocking M2 polarization of human macrophage by the hPSCs. The peptide was indeed capable of inhibiting hPSC-mediated M2 polarization of human macrophages ( Fig. 5g ). 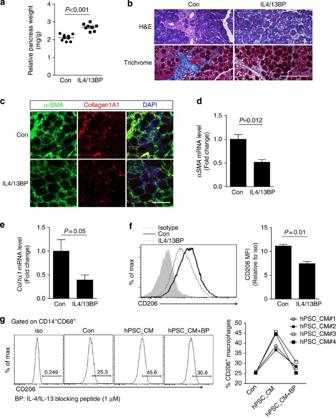Figure 5: IL-4/IL-13-blocking peptide ameliorates established CP. IL-4/IL-13-blocking peptide (IL4/13BP i.p., 50 μg per mouse ,5 days per week) was administrated to mice 2 weeks after starting CP induction and mice were killed as previous after 4 weeks of caerulein injections. (a) Relative pancreas weight from Con and IL4/13BP-treated mice are shown.n=8–9 per group, means±s.e.m. (unpaired two-tailed Student’st-test). (b) Representative of pancreas H&E and Trichrome staining. Scale bar, 200 μm. (c) Representative immunofluorescence images of the pancreas from indicated mice (co-stained with α-SMA, Collagen1A1 and DAPI). Scale bar: 50 μm. (d,e) RT–PCR analysis ofα-SMAandCol1α1(Collagen1A1) gene expression in the pancreas of indicated mice. Means±s.e.m. (unpaired two-tailed Student’st-test) (f) Flow cytometry analysis of CD206 expression (MFI) by pancreatic macrophages (CD11b+F4/80+) isolated from indicated mice. Means±s.e.m. (unpaired two-tailed Student’st-test). (g) Human macrophages as above were cultured with control medium (Con), conditioned medium from hPSCs (hPSC_CM) or hPSC_CM pretreated with 1 μM IL4/13BP (hPSC_CM+BP) for 24 h. Expression of CD206 (% CD206+macrophages) was analysed using flow cytometry. Figure 5: IL-4/IL-13-blocking peptide ameliorates established CP. IL-4/IL-13-blocking peptide (IL4/13BP i.p., 50 μg per mouse ,5 days per week) was administrated to mice 2 weeks after starting CP induction and mice were killed as previous after 4 weeks of caerulein injections. ( a ) Relative pancreas weight from Con and IL4/13BP-treated mice are shown. n =8–9 per group, means±s.e.m. (unpaired two-tailed Student’s t -test). ( b ) Representative of pancreas H&E and Trichrome staining. Scale bar, 200 μm. ( c ) Representative immunofluorescence images of the pancreas from indicated mice (co-stained with α-SMA, Collagen1A1 and DAPI). Scale bar: 50 μm. ( d , e ) RT–PCR analysis of α-SMA and Col1α1 (Collagen1A1) gene expression in the pancreas of indicated mice. Means±s.e.m. (unpaired two-tailed Student’s t -test) ( f ) Flow cytometry analysis of CD206 expression (MFI) by pancreatic macrophages (CD11b + F4/80 + ) isolated from indicated mice. Means±s.e.m. (unpaired two-tailed Student’s t -test). ( g ) Human macrophages as above were cultured with control medium (Con), conditioned medium from hPSCs (hPSC_CM) or hPSC_CM pretreated with 1 μM IL4/13BP (hPSC_CM+BP) for 24 h. Expression of CD206 (% CD206 + macrophages) was analysed using flow cytometry. Full size image Generally, CP is accepted as an irreversible and fibrotic disease, and current management is supportive at best with focus in controlling pain and complications associated with the exocrine and endocrine loss of functions [4] . Following the discovery and the central role of PSCs in pancreatic fibrosis, potential treatment approaches in CP have proposed inhibition or inactivation of PSCs [25] . However, the immune responses and immune cell contribution to PSC activation during CP progression remain poorly understood. In the current study, we explore the characteristics and role of macrophages, as well as aim to identify mechanisms for macrophage interaction with PSCs in CP. Our results show that AAMs play an important role in CP fibrogenesis and identify the key pathway that can be potentially targeted. Macrophages have been proposed as the master regulators of inflammation and fibrosis in diseases such as liver fibrosis and systemic sclerosis [9] . Our study reveals that macrophages are increased in both mouse and human CP. CP is also associated with an increase in macrophage-related cytokines and chemokines, supporting for a critical role of macrophages in disease progression. Since macrophages differentiate as well as polarize in tissues and do not recirculate, our data using competitive BM chimeras and proliferation studies suggest that both local ( in situ ) macrophage proliferation and monocyte recruitment contribute to the macrophage accumulation in CP. In sharp contrast to AP where M1 predominate, CP favoured alternative activation of macrophages. Macrophages represent a spectrum of activated phenotypes rather than a discrete stable subpopulation [26] , and it is possible that macrophages in different activation states or mixed phenotypes coexist as have been shown under different physiological and pathological conditions [27] . Indeed, these phenomena may account for the varied expression level of some of the M2 markers (for example, YM1 ). Macrophages in our CP model and those from PSC cocultures had higher mRNA expression of TGFβ and PDGFβ, suggesting possible role in directly promoting proliferation and activation of PSCs [6] , [28] , [29] . These macrophages express higher levels of tissue inhibitor metalloproteinase 2 ( TIMP2 ) and matrix metalloproteinase 9 ( MMP9 ) and thus may also regulate extracellular matrix turnover ( Fig. 2a ). Moreover, their expression of IL-10 and downregulation of MHCII suggest immunosuppressive properties. Several studies have documented macrophage plasticity with these cells switching from one functional phenotype to another in response to variable local microenvironmental signals [27] , [30] , [31] , [32] . In light of the central role of PSCs in CP progression, we took into account that the PSCs may be providing signals to maintain and facilitate the increased alternative activation observed in CP. In fact, relative to pro-inflammatory cytokines, PSCs (from both mouse and human pancreas) expressed higher levels of Th2 cytokines, IL-4 and IL-13, which are required for macrophage alternative activation [8] , [33] . Furthermore, using IL-4Rα-sufficient and -deficient mixed BM chimeras, we confirmed that IL-4Rα signalling is required for alternative activation of macrophages in CP. Both IL-R4α −/− and LysM cre IL-4Rα flox/flox mice had similar decreases in pancreatic fibrosis and PSC activation (α-SMA), suggesting that the contribution of IL-R4α signalling in fibrosis during CP is myeloid- or macrophage-dependent. IL-4/IL-13 −/− mice were even less susceptible to caerulein-induced CP. Similar to IL-4, IL-13 signals through the IL-4 receptor (a heterodimeric receptor composed of IL-4Rα and IL-13Rα1); however, IL-13 can also bind to IL-13Rα2 (which does not bind IL-4) to trigger downstream signals. IL-13 has been shown to be a major inducer of fibrosis in many chronic infectious and autoimmune diseases in part via the IL-13Rα2 (ref. 34 ). Inhibition of both IL-4 receptor and IL-13Rα2 signalling in the double knockout mice ( IL-4/IL-13 −/− ) as compared with inhibition of the IL-4 receptor only in the IL-4Rα −/− and LysM cre IL-R4α flox/flox mice may account for the increased protection against CP development observed in the IL-4/IL-13 −/− mice. Functional macrophage polarization is observed in vivo under physiological and pathological conditions [21] . The phenotype of polarized M1 or M2 macrophages can, to some extent, be reversed in vitro and in vivo [35] , [36] . Therefore, reorienting and reshaping macrophage polarization has been considered as a therapeutic strategy for several diseases. In our study, we attempted to reshape macrophage polarization through genetically deficient mice or via blocking IL-4/IL-13 by pharmacological means. Consistent with results from IL-4/IL-13-deficient mice, treatment with the IL-4/13-blocking peptide following induction of CP decreased macrophage alternative activation and ameliorated pancreatic fibrosis. This immune-based therapy in experimental CP challenges the thinking that CP cannot be actively treated, reversed or halted from progressing. Future studies determining the contribution of IL-4 versus IL-13 will be of interest to further define and design specific target(s). It is worth pointing out that some limitations still exist in correlating to human studies [22] : (1) limited availability of human CP tissues from surgical resections; (2) challenge of identification of equivalent macrophage subsets in humans because of lack of panels of markers. Despite these, our in vitro human PSCs and macrophage coculture experiments are consistent with the results obtained in mouse studies. We show that activated mouse and human PSCs secrete Th2 cytokines and enhance M2 polarization, leading to a potentially perpetual feed forward process ( Fig. 6 ). These findings are confirmed using IL-4Rα-deficient macrophages, and IL-4/IL-13-blocking peptide in experimental mouse and human systems. Interfering with IL-4Rα signalling and/or PSC activation is likely to turn off this feed forward process in CP. Our in vitro human studies, together with results observed from mouse studies, provide a proof-of-concept for potential targetable pathway and first step towards bench to bedside translation. 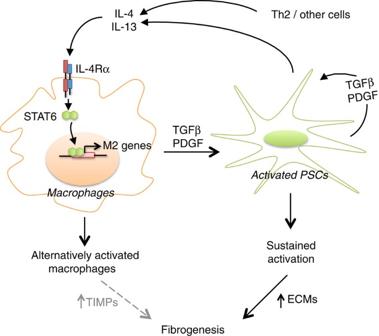Figure 6: Schematic representation of macrophage and pancreatic stellate cell (PSC) interation in chronic pancreatitis.  Figure 6: Schematic representation of macrophage and pancreatic stellate cell (PSC) interation in chronic pancreatitis. Full size image Mice BALB/c, C57BL/6, SJL, B6.SJL, IL-4Rα −/− , CCR2 KO mouse strains were purchased from Jackson Laboratory and bred in-house. LysM cre IL-4Rα flox/flox (ref. 24 ) and IL-4/IL-13 −/− (ref. 37 ) mice on BALB/c background were generated as described. All experimental mice were age- (6–8 weeks) and sex-matched, and animal experiments were approved by the Stanford University institutional animal care and use committees. Mixed bone marrow chimeras Competitive mixed BM chimeric mice were generated by lethally irradiating CCR2 WT CD45.1 + CD45.2 + C57BL/6 mice with 9.5-Gy γ radiation in two doses at ∼ 3 h apart, followed by i.v. injection of 5 × 10 6 BM cells comprising 1:1 mixture of cells from CCR2 WT CD45.1 + and CCR2 KO CD45.2 + mice. Chimeric mice were left to engraft for at least 8 weeks before further experimental manipulation. Pancreatitis model and treatment AP was induced with caerulein injection in mice as previously described [38] , [39] . CP was induced by repetitive caerulein injections [14] , [40] . In brief, mice were given six hourly intraperitoneal (i.p.) injections of 50-μg kg −1 body weight caerulein (Sigma-Aldrich) 3 days per week, for a total of 4 weeks. Mice were then killed and analysed 3 days after the last caerulein injection. For blocking peptide study all mice were given caerulein injection 3 days per week for a total of 4 weeks as above, and 2 weeks following start of the caerulein injection mice were either given vehicle control (PBS) or IL-4/IL-13-blocking peptide (50 μg per mouse, 100 μl daily for 5 days per week × 2 weeks) until being killed 4 weeks and 3 days later as above. Human samples Human pancreatic tissues from patients with CP, pancreatic ductal adenocarcinoma (PDAC) and normal pancreas margins from patients with PDAC, and one from a patient with normal pancreas (patient had adjacent nonpancreatic tumour that required partial resection of the pancreas) were obtained from the Stanford tissue bank with Local Ethics Committee approval and patient consents. Histology and immunofluorescence Mice were killed by CO 2 inhalation, and then their pancreata were rapidly removed. Pancreas pieces were immediately fixed in 10% formalin or frozen in Tissue-Tek OCT compound. Fixed tissues were sectioned and used for haemotoxylin and eosin and Trichrome staining (performed in the Histo-Tec Laboratory). Frozen tissues were also sectioned for immunofluorescence staining with indicated antibodies and analysed with confocal microscopy. The Luminex assay The assay was performed in the Human Immune Monitoring Center at Stanford University [39] . Human 63-plex or Mouse 26 plex kits were purchased from Affymetrix and used according to the manufacturer’s recommendations with modifications as described below. Briefly, samples were mixed with antibody-linked polystyrene beads on 96-well filter-bottom plates and incubated at room temperature for 2 h followed by overnight incubation at 4 °C. Room temperature incubation steps were performed on an orbital shaker at 500–600 r.p.m. Plates were vacuum-filtered and washed twice, and then incubated with biotinylated detection antibody for 2 h at room temperature. Samples were then filtered and washed twice as above and resuspended in streptavidin-phycoerythrin (PE). After incubation for 40 min at room temperature, two additional vacuum washes were performed and the samples resuspended in Reading Buffer. Each sample was measured in duplicate. Plates were read using a Luminex 200 instrument. Antibodies and flow cytometry All antibodies used for flow cytometry were purchased from Biolegend, unless indicated. For surface staining, murine cells were stained with the following antibodies: APC-CD45.2 (109814, 1:200), PE/Cy7-CD4 (100528, 1:300), Percp/Cy5.5-CD11b (101228, 1:200), BV421-F4/80 (123137, 1:200), APC/Cy7-CD11C (117324, 1:200), PE-IL-4Rα (144803 1:100), AF488-CD206 (141710, 1:100), AF700-MHCII (107622, 1:300), PB-Ly6C (128014, 1:200), PE/Cy7-Ly-6G (127617, 1:300), PE-FcɛRIα (134307, 1:200), AF488-ckit (105815, 1:200), APC-eFluor780-CD45.1 (47-0453-82, eBioscience, 1:200) and PE-Siglec-F (562068, BD Biosciences, 1:200). Human cells were stained with PE/Cy7-CD14 (301814,1:100), AF488-CD206 (321114, 1:50) and APC-CD68 (333810, 1:100). For intracellular cytokine staining, cells were activated with phorbol myristate acetate (50 ng ml −1 ) and ionomycin (1 μg ml −1 ), in the presence of brefeldin A (10 μg ml −1 , eBioscience) for 4 h at 37 °C before staining. The cells were then fixed and permeabilized using the eBioscience kit following the manufacturer’s guidelines. APC-IL10 (554468, 1:100) and isotype control (556924, 1:100) from BD Biosciences were used for intracellular staining. For intracellular TNFα staining, cells were incubated with or without lipopolysaccharide (100 ng ml −1 , InvivoGen) in the presence of brefeldin A before surface-staining. PE-TNFα (554419, 1:200) and isotype control (554685, 1:200) from BD Biosciences were used. For detection of intracellular Ki-67 and BrdU, cells were stained for surface makers and then fixed and permeabilized using Foxp3 staining buffer set (eBioscience). For BrdU staining, cells were first incubated with DNase for 1 h at 37 °C. The Cells were then stained with PE–BrdU (339812, 1:100) or AF488-Ki67 (558616, BD Biosciences, 1:50). Dead cells were excluded from analysis using violet viability stain (Invitrogen). Flow cytometry data collection was performed on Fortessa LSRII (BD Biosciences) and analysed using the FlowJo software (Tree Star Inc.). Cell preparation and in vitro cultures Pancreatic leukocytes were isolated using collagenase digestion method described previously for flow cytometry analysis [38] . PSCs from CP mice were isolated by outgrowth method as described [41] . Primary human PSCs from normal margins and PDAC were isolated using gradient centrifugation and outgrowth method, respectively [41] , [42] . Murine PSCs were cultured in DMEM/F12 (1:1) medium containing 10% FBS. Where indicated, mouse PSCs were cultured with TGFβ (5 ng ml −1 ), PDGFβ (10 ng ml −1 ) or media control for 6 h before being collected for mRNA and qPCR analyses. Human PSCs were cultured in IMDM medium containing 20% FBS. Isolated PSCs were ready for use after the second passage. Conditioned medium (CM) from the PSC was collected after 2 days of culture and when cells reached 70–80% confluence. The CM was centrifuged to remove cellular debris before use. BMDMs were prepared as previously described [39] . For human monocyte-derived macrophage preparation, human peripheral blood mononuclear cells were isolated from buffy coat using Ficoll-Hypaque density gradient centrifugation, and then monocytes were further enriched by CD14 + magnetic beads (Miltenyi Biotec). Enriched monocytes were cultured with complete RPMI medium containing 50 ng ml −1 human macrophage CSF. On day 6, human macrophages are ready for use [43] . PSC and BMDM coculture experiments were performed in the Transwell system (Corning) in the DMEM/F12 medium with 10% FBS. After seeding 5 × 10 4 PSCs in the bottom well, 5 × 10 5 BMDMs were seeded on the upper mesh (pore size: 0.4 μm). Macrophages were collected for analysis after 48 h of the coculture. Quantitative RT–PCR Th pancreas or cells were lysed with Trizol reagent (Invitrogen) for total RNA preparation according to the manufacturer’s instructions. Briefly, cDNA was generated using the GoScript reverse transcription system (Promega). Quantitative PCR was performed with an ABI-7900 Sequence Detection System (Applied Biosystems) using designed specific TaqMan probes and primers as follows: YM1 (Forward, 5′- TGGTGAAGGAAATGCGTAAA -3′; reverse, 5′- GTCAATGATTCCTGCTCCTG -3′; probe, 5′- AGCAGCCTTGGAATGTCTTTCTCCA -3′); FIZZ1 (forward, 5′- AGGAACTTCTTGCCAATCCA -3′; reverse, 5′- ACAAGCACACCCAGTAGCAG -3′; probe, 5′- CCTCCTGCCCTGCTGGGATG -3′); □rg1 (forward, 5′- AGACCACAGTCTGGCAGTTG -3′; reverse, 5′- CCACCCAAATGACACATAGG -3′; probe, 5′- AAGCATCTCTGGCCACGCCA -3′); CD206 (forward, 5′- TGATTACGAGCAGTGGAAGC -3′; reverse, 5′- GTTCACCGTAAGCCCAATTT -3′; probe, 5′- CACCTGGAGTGATGGTTCTCCCG -3′); CD301 (forward, 5′- ACTGAGTTCCTGCCTCTGGT -3′; reverse, 5′- ATCTGGGACCAAGGAGAGTG -3′; probe, 5′- CACTGCTGCACAGGGAAGCCA -3′); IL-10 (forward, 5′- CCCAGAAATCAAGGAGCATT -3′; reverse, 5′- TCACTCTTCACCTGCTCCAC -3′; probe, 5′- TCGATGACAGCGCCTCAGCC -3′); TGFβ (forward, 5′- CCCTATATTTGGAGCCTGGA -3′; reverse, 5′- CTTGCGACCCACGTAGTAGA -3′; probe, 5′- CCGCAGGCTTTGGAGCCACT -3′); inducible nitric oxide synthase (forward, 5′- ACCTTGTTCAGCTACGCCTT -3′; reverse, 5′- TCTTCAGAGTCTGCCCATTG -3′; probe, 5′- TGCTCCTCTTCCAAGGTGCTTGC -3′); TNFα (forward, 5′- CCAAAGGGATGAGAAGTTCC -3′; reverse, 5′- CTCCACTTGGTGGTTTGCTA -3′; probe, 5′- TGGCCCAGACCCTCACACTCA -3′); αSMA (forward, 5′- CTCCCTGGAGAAGAGCTACG -3′; reverse, 5′- TGACTCCATCCCAATGAAAG -3′; probe, 5′- AAACGAACGCTTCCGCTGCC -3′); Collegen1A1 (forward, 5′- AGAAGGCCAGTCTGGAGAAA -3′; reverse, 5′- GAGCCCTTGAGACCTCTGAC -3′; probe, 5′- TGCCCTGGGTCCTCCTGGTC -3′); Fibronectin (forward, 5′- TGGTGGCCACTAAATACGAA -3′; reverse, 5′- GGAGGGCTAACATTCTCCAG -3′; probe, 5′- CAAGCAGACCAGCCCAGGGA -3′); TIMP1 (forward, 5′- CCAGAAATCAACGAGACCAC -3′; reverse, 5′- GGCATATCCACAGAGGCTTT -3′; probe, 5′- TCTGCGGCATTTCCCACAGC -3′); MMP9 (forward, 5′- TCCTTGCAATGTGGATGTTT -3′; reverse, 5′- CTTCCAGTACCAACCGTCCT -3′; probe, 5′- TGCAGAGCGCCCTGGATCTC -3′); GAPDH (forward, 5′- TGTGTCCGTCGTGGATCTGA -3′; reverse, 5′- CCTGCTTCACCACCTTCTTGA -3′; probe, 5′- CCGCCTGGAGAAACCTGCCAAGTATG -3′). Samples were normalized to GAPDH and displayed as fold induction over untreated controls, unless otherwise stated. Statistical analysis Unpaired Student’s t -test was used to determine statistical significance, unless otherwise indicated, and P value of less than 0.05 was considered significant. Where indicated, one-way analysis of variance and Tukey’s post hoc test was used as described in figure legend. Values are expressed as mean±s.e.m. (Prism 5; GraphPad Software). Unless indicated, results are from at least three independent experiments. How to cite this article : Xue, J. et al . Alternatively activated macrophages promote pancreatic fibrosis in chronic pancreatitis. Nat. Commun. 6:7158 doi: 10.1038/ncomms8158 (2015).